How intermolecular geometrical disorder affects the molecular doping of donor–acceptor copolymers Molecular doping of conjugated polymers represents an important strategy for improving organic electronic devices. However, the widely reported low efficiency of doping remains a crucial limitation to obtain high performance. Here we investigate how charge transfer between dopant and donor–acceptor copolymers is affected by the spatial arrangement of the dopant molecule with respect to the copolymer repeat unit. We p-dope a donor–acceptor copolymer and probe its charge-sensitive molecular vibrations in films by infrared spectroscopy. We find that, compared with a related homopolymer, a four times higher dopant/polymer molar ratio is needed to observe signatures of charges. By DFT methods, we simulate the vibrational spectra, moving the dopant along the copolymer backbone and finding that efficient charge transfer occurs only when the dopant is close to the donor moiety. Our results show that the donor–acceptor structure poses an obstacle to efficient doping, with the acceptor moiety being inactive for p-type doping. Recently, a wide range of new applications for doped polymers has emerged, which include thermoelectrics [1] , [2] , spintronics [3] , (opto)electronics [4] and biosensors [5] . This recent progress was mainly driven by the design of robust molecular dopants [6] , which when mixed with the semiconductor in controlled amounts can finely tune the electrical characteristics of the material. Despite the increasing interest in device applications, there is only limited understanding of how molecular doping of conjugated polymers occurs. Doping organic semiconductors is different in nature with respect to the similar concept applied in inorganic semiconductor technology. While p- and n-type doping of silicon, for example, by boron or phosphor, respectively, means the substitution of atoms in a covalently bound lattice, molecular doping of conjugated polymers generally refers to charge transfer occurring between molecular components in a film. The molecules form a van der Waals solid and each molecule retains its chemical identity. This intermolecular type of doping opens the possibility for many different geometrical configurations, exhibiting different degrees of electronic interaction and resulting in a variation in doping efficiency as we demonstrate in this article. In our work, we discuss the doping efficiency referring to the amount of charge transferred between the dopant and the conjugated polymer. To achieve p- or n-type molecular doping, highly electronegative or highly electron donating molecules are mixed in low concentration with an organic semiconductor [6] . The most striking success of this approach is the realization of organic field effect transistors with improved operational stability [4] , [7] , highly efficient organic light emitting diodes [8] , [9] and solar cells with improved performance [10] , [11] . We focus on the case of p-type doping, that is, the introduction of excess positive charge carriers (holes) in the semiconductor. In this respect, the most commonly presented picture is the ground-state transfer of one electron from the highest occupied molecular orbital (HOMO) of the polymer to the lowest unoccupied molecular orbital (LUMO) of the electronegative dopant molecule [6] , [12] . Holes in the semiconductor increase the carrier density, leading to an enhancement of the electrical conductivity. Furthermore, it has been recently reported by several groups that doping can fill trap states, resulting in improved carrier mobility in different types of device architectures [7] , [10] , [13] , [14] . However, these beneficial effects are difficult to reliably control. The density of free carriers and the dopant density in the semiconductor, thus the efficacy of the charge transfer process, are the most discussed variables in the parameters space [12] , [15] . Particularly interesting are the recent observations showing evidence that the effect of doping on conductivity enhancement in donor–acceptor (D–A) copolymers is lower than that for homopolymers [16] . D–A copolymers have revolutionized the field of organic electronics by showing single-junction solar cells reaching close to 10% power conversion efficiency [17] , carrier mobility >10 cm 2 V −1 s −1 in field effect transistors [18] and bipolar transport [19] . The most important feature of D–A copolymers is the possibility of finely tuning the energy bandgap via the selection of the two moieties [20] . The intrinsically more complex structure of the repeat unit of D–A copolymers, however, brings more difficulties to the microscopic description of doping in these systems. Studies aiming for a microscopic description of doping have appeared recently mainly focusing on homopolymers [12] , [21] , [22] , [23] , [24] , [25] , leaving the challenge of describing the interaction between dopants and D–A alternating copolymers largely unaddressed. A detailed understanding of the mechanism of doping is needed in order to shed light on the very low amount of free charges per dopant (~4 charges donated every 100 dopants) observed in D–A copolymers [26] , and offer a solid understanding for future materials development. In this article, we provide a microscopic description of doping in the D–A copolymer (poly[2,6-(4,4-bis(2-ethylhexyl)-4H-cyclopenta[2,1-b;3,4-b′′]dithiophene)- alt -4,7-(2,1,3-benzothiadiazole)] (PCPDT-BT) mixed at different concentrations with the dopant 2,3,5,6-tetrafluoro-7,7,8,8-tetracyanoquinodimethane (F4-TCNQ). In PCPDT-BT, the cyclopenta-dithiophene (CPDT) moiety is D and the BT moiety is A. We used infrared spectroscopy to study microscopic changes induced by doping, as this technique is known to be sensitive to the presence of charged species in conjugated polymers through molecular vibrations [27] , [28] , [29] . An advantage of looking at vibrations is that their absorption resonances are less affected by inhomogeneous broadening, an effect which is instead markedly impacting the amount of information possibly extracted from electronic transitions in conjugated polymers [30] , [31] . In contrast to previous studies looking at the vibrational absorption bands of the dopant [21] , [32] , our work is concentrating on the modes of the conjugated polymer backbone. This distinctive approach is motivated by the following two reasons: (i) the much higher sensitivity of these bands in witnessing charge carriers and thus the possibility to study the low doping concentration regime of 1% molar ratio, and (ii) a more detailed understanding of the role of polymer-dopant geometrical structure on doping, which we achieve by ab initio simulations despite the demanding computational effort in reproducing the experimental spectra. We demonstrate that if the dopant molecule is close to the A moiety of the copolymer, there is no efficient charge transfer. This can, therefore, be considered as an inactive site, lowering the overall efficiency of doping in the semiconductor film. Efficient charge transfer is instead observed for F4-TCNQ close to D. The critical aspect of intermolecular geometrical disorder is further demonstrated by a series of experiments with the homopolymer PCPDT, which contains only D in the repeat unit. As expected in the case of more efficient doping, this homopolymer exhibits the characteristic spectroscopic signals of charges on the conjugated chain at lower doping concentrations. FTIR spectroscopy on doped polymer films In Fig. 1a , the chemical structures of the copolymer PCPDT-BT, the homopolymer PCPDT and the dopant F4-TCNQ are shown. Figure 2a shows the Fourier transform infrared (FTIR) spectra of PCPDT-BT in the pristine form (0%) and doped with F4-TCNQ at different % molar ratios. 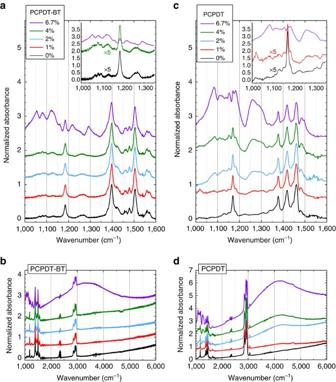Figure 2: FTIR absorption spectra of doped thin films. Normalized FTIR absorption spectra in the region of backbone vibrations for (a) PCPDT-BT and (c) PCPDT spin-coated thin films, pristine and doped with F4-TCNQ in different molar percentages (see legend). The molar percentage is calculated using the number of moles of F4-TCNQ divided by the number of moles of polymer repeat unit. The insets ina,care a zoom of the low wavenumber part, with the intensity of neutral and doped samples spectra (4% and 1% for PCPDT-BT and PCPDT, respectively) multiplied five times to better compare the 6.7% samples. (b,d) Wider wavenumber ranges for PCPDT-BT and PCPDT, respectively. All the spectra are normalized on the band peaked atca. 1,400 cm−1for PCPDT-BT samples and atca. 1,460 cm−1for PCPDT, and offset for clarity. Inb,d, the light scattering contribution to the baseline was not corrected. The vibrational bands in the 2,800–3,000 cm−1region originate from the alkyl side chains of the polymers. F4-TCNQ vibrations, either in neutral or charged state51, are not apparent due to the low dopant concentrations. Each spectrum is normalized to the absorbance of the band peaked at 1,400 cm −1 . To calculate the % molar ratio, we use the number of moles of F4-TCNQ divided by the number of moles of polymer repeat unit. Using this definition, 4% molar ratio corresponds to 25 polymer repeat units for each F4-TCNQ molecule. The spectra of doped samples with molar ratio >4% exhibit additional infrared active vibrational modes in the region 1,000–1,300 cm −1 , which are almost undetectable in pristine PCPDT-BT. By zooming this spectral region in the inset, we note a remarkable increase in the absorption intensity of modes at 1,055, 1,080 and 1,120 cm −1 in comparison with the one at 1,190 cm −1 , as the dopant molar ratio is increased to 6.7%. The high intensity vibrational bands of pristine PCPDT-BT in the region 1,360–1,550 cm −1 are present in all samples introduced in this figure and do not exhibit any detectable change in spectral position. We attribute the intensity enhancement of absorption between 1,000 and 1,300 cm −1 to the presence of dopant-induced hole polarons on the polymer chain. The high oscillator strength for vibrational absorption bands in presence of charged states has been extensively documented in conjugated molecules [27] , [33] , [34] . Figure 2b shows the infrared spectra on a larger spectral range up to 6,000 cm −1 for the same PCPDT-BT samples presented above. These cover not only the region of fingerprint molecular vibrations but also the polaronic transitions due to the hole polarons on the conjugated segments of the copolymer. 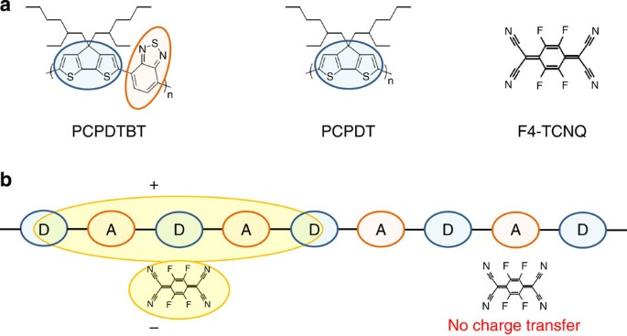Only at 6.7%, we observe the appearance of a prominent polaron band centred at 3,500 cm −1 . Figure 1: Chemical structures. (a) Structure of the D–A copolymer PCPDT-BT, the homopolymer PCPDT and the dopant F4-TCNQ. The light blue and orange ovals highlight the donor (D) and acceptor (A) moieties of the repeat unit, respectively. (b) Scheme showing the dependence of electron transfer efficiency on the position of F4-TCNQ molecules along the D–A chain; when F4-TCNQ is on theDmoiety, electron transfer is efficient, and when on the A moiety there is no charge transfer. Figure 1: Chemical structures. ( a ) Structure of the D–A copolymer PCPDT-BT, the homopolymer PCPDT and the dopant F4-TCNQ. The light blue and orange ovals highlight the donor (D) and acceptor (A) moieties of the repeat unit, respectively. ( b ) Scheme showing the dependence of electron transfer efficiency on the position of F4-TCNQ molecules along the D–A chain; when F4-TCNQ is on the D moiety, electron transfer is efficient, and when on the A moiety there is no charge transfer. Full size image Figure 2: FTIR absorption spectra of doped thin films. Normalized FTIR absorption spectra in the region of backbone vibrations for ( a ) PCPDT-BT and ( c ) PCPDT spin-coated thin films, pristine and doped with F4-TCNQ in different molar percentages (see legend). The molar percentage is calculated using the number of moles of F4-TCNQ divided by the number of moles of polymer repeat unit. The insets in a , c are a zoom of the low wavenumber part, with the intensity of neutral and doped samples spectra (4% and 1% for PCPDT-BT and PCPDT, respectively) multiplied five times to better compare the 6.7% samples. ( b , d ) Wider wavenumber ranges for PCPDT-BT and PCPDT, respectively. All the spectra are normalized on the band peaked at ca . 1,400 cm −1 for PCPDT-BT samples and at ca . 1,460 cm −1 for PCPDT, and offset for clarity. In b , d , the light scattering contribution to the baseline was not corrected. The vibrational bands in the 2,800–3,000 cm −1 region originate from the alkyl side chains of the polymers. F4-TCNQ vibrations, either in neutral or charged state [51] , are not apparent due to the low dopant concentrations. Full size image We contrast these results on the copolymer with the spectra for the pristine and doped homopolymer. Figure 2c shows normalized infrared spectra of PCPDT in the same spectral interval and same F4-TCNQ molar concentrations of Figure 2a . The absorption intensity increases in the region from 1,000 to 1,300 cm −1 as a function of doping and it is evident at molar percentages lower than those reported above for the copolymer PCPDT-BT. Prominent vibrational bands are at 1,083, 1,108 and 1,182 cm −1 , together with a broad structure of bands from 1,225 to 1,335 cm −1 . Importantly, here the effect of doping is visible already at 1% F4-TCNQ molar concentration, with a detectable enhancement of the broad band between 1,225 and 1,325 cm −1 (inset Fig. 2c ). At 2%, the effect becomes more substantial with the enhancement of bands in the region between 1,000 and 1,200 cm −1 as well. The spectrum of pristine PCPDT (lower black curve in main panel) is characterized by four intense vibrational bands at 1,165, 1,378, 1,418 and 1,460 cm −1 . These four vibrational transitions are present in all the samples that we show. Increasing the dopant concentration in PCPDT films also results in a vibrational band at 1480, cm −1 which gains intensity with dopant concentration. This is in contrast to the spectra of doped PCPDT-BT ( Fig. 2a ), where the 1,350 to 1,600-cm −1 part of the spectrum remains almost unchanged upon doping. Figure 2d shows the enlarged spectral range with the polaronic transition peaking at ~4,100 cm −1 . In agreement with the intensity trend in the vibrational bands, also the polaronic transition of PCPDT appears at lower molar concentration with respect to what we observe in the copolymer. Interestingly, the polaronic absorption band of PCPDT can be clearly distinguished only for dopant percentages >2%, whereas signatures of doping enhanced vibrational bands are seen at lower concentrations of 1% as presented above. This latter observation indicates that the enhancement of oscillator strength (intensity) of certain vibrational transitions allows for a more sensitive monitoring of charged states with respect to the polaronic transitions solely. Ab initio simulations of vibrational spectra using DFT We now focus on the theoretical description of the infrared spectra in the region of the conjugated backbone vibrations, that is, 800–1,600 cm −1 . Spectra are shown as integrated infrared absorption intensity as a function of frequency (see Methods section for details on calculations). 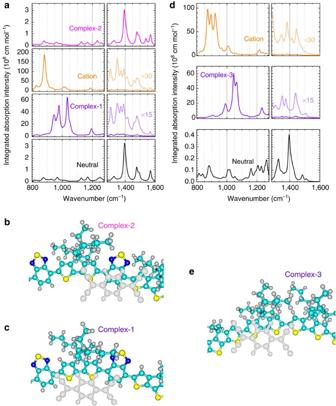Figure 3: Vibrational spectra calculated by DFT. Calculated vibrational spectra of (a) PCPDT-BT and (d) PCPDT in different configurations as indicated by the labels in the graphs. The ordinates are in units of integrated absorption intensity (see Methods section). Each spectrum is divided in the following two parts: for wavenumbers <1,280 cm−1thexaxis has not been scaled, whereas for wavenumbers >1,280 cm−1a scaling factor of 0.935 has been applied. To show some of the weaker absorption bands on the same scale, part of the spectra of Complex-1 and Complex-3 has been multiplied by 15 and part of the spectra of the cations has been multiplied by 30. (b,c,e) Image cuts of the optimized molecular geometries used to calculate the spectra of Complex-2, Complex-1 and Complex-3, respectively. The F4-TCNQ molecule lies in front of the polymer and is coloured in grey for better visualization. Figure 3a shows the computed vibrational spectrum for a polymer strand of PCPDT-BT made of four and a half repeat units (structure in Supplementary Fig. 1 ) simulated with a continuum model of the surrounding medium defined by the bulk dielectric constant [35] . The computed spectrum (lower black curve) reproduces with a good agreement the experimental features observed in Fig. 2a for pristine PCPDT-BT. We note that there is also a reasonable agreement in the prediction of the relative intensities of the vibrational bands. The peak at 1,397 cm −1 is reproduced as the most intense followed by the peaks in the region close to 1,500 cm −1 and the one at 1,568 cm −1 . Following a standard procedure described in the Methods section, we scaled the calculated frequencies by a factor <1 in the part of the spectra >1,280 cm −1 (ref. 36 ). Figure 3a shows also the spectrum of Complex-1, a molecular cluster obtained by energetically optimizing the geometry of F4-TCNQ in proximity of one of the CPDT moieties of PCPDT-BT ( Fig. 3c ). The computed infrared spectrum has changed markedly compared with the neutral copolymer strand and exhibits intense vibrational bands in the region from 1,000 to 1,200 cm −1 . We point out that the band peaked at 1,033 cm −1 of Complex-1 carries a 20 times larger intensity than the most intense peak of the neutral copolymer at 1,397 cm −1 . This appears to be qualitatively consistent with the charge-induced intensity enhancement that we experimentally observed. In Fig. 3a , we also show the following two additional spectra: the copolymer without F4-TCNQ, but with a positive charge on the chain strand, that is, a cation, and Complex-2, which is a different optimized geometry where the dopant F4-TCNQ is in the vicinity of the A moiety ( Fig. 3b ). The computed spectrum of the cation resembles Complex-1 in terms of intensity of the bands and similarity of the enhanced modes ( Supplementary Figs 2 and 3 ). Complex-2 has, instead, a spectrum almost identical to the neutral copolymer. Further, the Mulliken analysis of partial charge density (see Methods section) indicates an almost complete charge transfer in Complex-1 (0.93 e on the polymer) and almost zero (−0.02 e on the polymer) in Complex-2. The similar enhancement of vibrational transitions in the region 800–1,200 cm −1 for the cation and Complex-1 spectra, together with the Mulliken charge density distribution, confirms that for F4-TCNQ on the D moiety charge transfer occurs and a hole polaron is formed, whereas with the F4-TCNQ on the A moiety charge transfer and polaron formation are hindered. Figure 3: Vibrational spectra calculated by DFT. Calculated vibrational spectra of ( a ) PCPDT-BT and ( d ) PCPDT in different configurations as indicated by the labels in the graphs. The ordinates are in units of integrated absorption intensity (see Methods section). Each spectrum is divided in the following two parts: for wavenumbers <1,280 cm −1 the x axis has not been scaled, whereas for wavenumbers >1,280 cm −1 a scaling factor of 0.935 has been applied. To show some of the weaker absorption bands on the same scale, part of the spectra of Complex-1 and Complex-3 has been multiplied by 15 and part of the spectra of the cations has been multiplied by 30. ( b , c , e ) Image cuts of the optimized molecular geometries used to calculate the spectra of Complex-2, Complex-1 and Complex-3, respectively. The F4-TCNQ molecule lies in front of the polymer and is coloured in grey for better visualization. Full size image With a similar approach to the one used for PCPDT-BT, we have computed the infrared spectra for the homopolymer PCPDT. Figure 3d shows a series of spectra for a PCPDT polymer strand of six repeat units in its neutral form, a complex with F4-TCNQ (named Complex-3) and the same strand without the dopant, but with a net positive charge representing a cation. The calculated spectrum for the neutral polymer (lower black curve in Fig. 3d ) has the highest intensity bands in the 1,300 to 1,500-cm −1 region, similar to the experimental one ( Fig. 2c ). The spectra of Complex-3 and of the cation show vibrational modes with high intensity in the low wavenumber region (800–1,300 cm −1 ), with intensities comparable to those of the copolymer PCPDT-BT. As already noted for the PCPDT-BT case, the similarity in spectral evolution of complex and cation testifies the transfer of one electron from the HOMO of the polymer to the LUMO of F4-TCNQ. The illustration of a selection of vibrational modes is shown in the Supplementary Figs 1–4 and 7–9 for PCPDT-BT and PCPDT, respectively. In addition Supplementary Figs 5, 6 and 10, 11 contain the assignment of some of the experimental bands to the calculated vibrational modes. The criteria used in the selection are described in the Supplementary Discussion . The most immediate message that can be drawn from our theoretical results is that the primary step in doping of conjugated copolymers is extremely sensitive to geometrical intermolecular disorder. If F4-TCNQ forms a complex where it is co-facially aligned with the CPDT moiety, D, electron transfer occurs and a segment of the copolymer chain becomes doped with a hole. In contrast, if F4-TCNQ is closer to the BT moiety, A, only a negligible amount of charge transfer occurs. This conclusion is schematically depicted in Fig. 1b and is further supported by the results on the homopolymer; here different geometrical configurations were tested ( Supplementary Fig. 13 and the Supplementary Discussion ). We found that charge transfer occurs with similar amounts of transferred charge (>0.90 e ), independent of the exact position of F4-TCNQ along the polymer backbone and with respect to the repeat unit. From calculations, we have estimated the difference in the total Gibbs energy between Complexes-1 and -2 ( Supplementary Table 1 ). This is ~0.22 eV, which is above thermal energy at room temperature. While this could imply an instability of Complex-2 in conditions of thermodynamic equilibrium, we stress that the preparation of films by spin coating is a kinetic out of equilibrium process. Thus, intermolecular arrangements such as the one of Complex-2 are likely to be present, with large potential barriers for reorganization [37] . In addition, this energy estimation is for two molecules, while in the film additional polymer chains in proximity could further stabilize the geometry of Complex-2. The calculations on PCPDT-BT:F4-TCNQ in Complex-1 geometry can be considered as an idealized realization of an effectively doped copolymer film, where each F4-TCNQ molecule in every four and a half repeat units is accepting an electron and generating a hole. The spectrum of such a hypothetical film should be largely dominated by the bands between 1,000 and 1,200 cm −1 ( Fig. 3a ). Furthermore, the region 1,300–1,600 cm −1 should show additional vibrational transitions of comparable intensity to the peak at 1,400 cm −1 , which are not present in the neutral copolymer strand. Note that the calculated absorption intensity for modes in this region are very similar for Complex-1 and neutral PCPDT-BT ( Fig. 3a ). In contrast to these predictions, for all the dopant concentrations that we have used in the PCPDT-BT films ( Fig. 2a ) we observe only the molecular vibrations characteristic of the pristine copolymer left (1,350–1,600 cm −1 ). Even at the highest molar percentage of 6.7%, the vibrational bands between 1,350 and 1,600 cm −1 remain the most intense with just an additional background on the red side of the 1,400-cm −1 peak. This dopant percentage would correspond to one F4-TCNQ every 15 repeat units, which is a situation comparable to our theoretical simulations of one in every four and half repeat units. This discrepancy between experiments and predictions based on density functional theory (DFT) simulations can be rationalized, considering that the absorption spectra of our doped thin films contain a superimposition of contributions from charged and neutral polymer strands, with the latter dominating. The question is then why a considerable amount of polymer strands (chromophores) appears to be left undoped even when, as argued above, the amount of F4-TCNQ molecules in the 6.7% film should be just a factor of ~3 away from what is required for charging a conjugated segment. In principle, F4-TCNQ could phase segregate in the film. Without being in contact with PCPDT-BT chains, some dopant molecules would be excluded from the doping process. At the low concentrations that we explore here, this is unlikely and dopant segregation would appear as saturation or decrease in the intensity of the polaronic absorption [38] , which we do not observe in any of our samples. Our computational investigations suggest a different explanation: even if F4-TCNQ is molecularly dispersed, there are some intermolecular configurations that do not lead to doping. The latter case is theoretically reproduced by the simulations with the dopant on the A unit (Complex-2 in Fig. 3c ). On one hand, it is important that doped polymer layers in devices are prepared with molecularly dispersed dopants. On the other hand, it is apparent from our work that even taking care of morphology issues, F4-TCNQ may find a stable configuration close to the A moiety, forming a very weak charge transfer complex that does not contribute to doping. This analysis is supported by the data and simulations on the homopolymer, which has a similar energy of the HOMO with respect to PCPDT-BT (see Methods section), and thus a very similar driving force for charge transfer, but exhibits doping characteristics at much lower F4-TCNQ concentration. Note that the absorption intensities of vibrational modes enhanced by charges are very similar for Complexes-1 and -3, and thus spectral features should appear at equal experimental concentrations if the doping efficiency was the same for both polymers. To summarize, our results reveal that intermolecular geometrical disorder acts as an intrinsic limitation to efficient doping of D–A-conjugated copolymers with F4-TCNQ, even in the case of homogeneous dopant dispersion in the film. There is a complementary important aspect on which our results can shed light and contribute to the microscopic understanding of doping in conjugated copolymers, that is, the degree of delocalization of the dopant-induced hole on the conjugated polymer. This is intrinsically correlated to the density of free carriers and charge carrier transport characteristics. Holes generated on the polymer backbone may remain localized in the proximity of the ionized dopant and thus exhibit a low probability of escaping from the Coulomb potential generated by the negative charge on the F4-TCNQ. In contrast, delocalized holes should have a larger probability of escaping the Coulomb potential by hopping on nearest neighbour conjugated chains and becoming mobile. Since the vibrational spectra and their description are particularly sensitive to the length of chemical bonds along the π-conjugated backbone, we could extract information on the polaron delocalization. We analysed the evolution of the C–C bond lengths along the PCPDT-BT copolymer strands in the neutral and charged states, as computed in our DFT calculations. As previously shown, the presence of a polaron on a conjugated polymer backbone is accompanied by an evolution from aromatic to quinoid structure [39] . 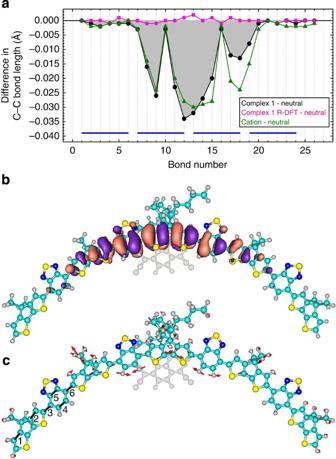Figure 4: Bond length alternation and mode visualization for Complex-1 (a) Difference between the calculated carbon–carbon (C–C) bond lengths of PCPDT-BT in Complex-1 and the neutral PCPDT-BT strand (black). The bond length difference compared with the neutral strand is shown also for PCPDT-BT in Complex-1 configuration calculated with R-DFT (pink) and for the PCPDT-BT cation (green). The line connecting the symbols is a guide to the eye. The C–C length of bond number 1 in the neutral chain is 1.421 Ångstrom. The bond numbering is defined as indicated by the black bars and labels on the first repeat unit inc. The blue horizontal bars indicate the polymer repeat units. (b) Molecular orbital of the positive polaron induced on the PCPDT-BT chain by charge transfer to F4-TCNQ. (c) Scaled vectors representing the vibrations corresponding to the absorption peaked at 1,033 cm−1(Fig. 3a) as calculated for Complex-1. For visual clarity, inb,c, the F4-TCNQ molecule lies behind the polymer chain. Figure 4a shows the difference between a selection of C–C bond lengths in the Complex-1 configuration and the same bonds in the neutral PCPDT-BT strand. These are the bonds mostly affected by the presence of a polaron. The convention used for the bond numbering is indicated in Fig. 4c . The change in bond length is up to 0.035 Å and it extends over two repeat units in front of the F4-TCNQ molecule. The main distortion (change in C–C length >0.01 Å) is over ~2 nm along the chain. Figure 4b shows the molecular orbital describing the polaron, that is, the singly occupied HOMO. By comparing Fig. 4a and Fig. 4b , the correlation between the change in bond length and the spatial extension of the polaron is apparent. In order to exclude any role of steric hindrance effects due to F4-TCNQ on the copolymer structure, Fig. 4a also shows the bond length change for Complex-1 geometry calculated using a restricted DFT (R-DFT) approach (see Methods section), where no charge is transferred and the C–C distances remain essentially the same as for the neutral copolymer. Figure 4: Bond length alternation and mode visualization for Complex-1 ( a ) Difference between the calculated carbon–carbon (C–C) bond lengths of PCPDT-BT in Complex-1 and the neutral PCPDT-BT strand (black). The bond length difference compared with the neutral strand is shown also for PCPDT-BT in Complex-1 configuration calculated with R-DFT (pink) and for the PCPDT-BT cation (green). The line connecting the symbols is a guide to the eye. The C–C length of bond number 1 in the neutral chain is 1.421 Ångstrom. The bond numbering is defined as indicated by the black bars and labels on the first repeat unit in c . The blue horizontal bars indicate the polymer repeat units. ( b ) Molecular orbital of the positive polaron induced on the PCPDT-BT chain by charge transfer to F4-TCNQ. ( c ) Scaled vectors representing the vibrations corresponding to the absorption peaked at 1,033 cm −1 ( Fig. 3a ) as calculated for Complex-1. For visual clarity, in b , c , the F4-TCNQ molecule lies behind the polymer chain. Full size image We have attempted to visualize the impact of Coulomb interactions on the polaron wavefunction delocalization. This is done by comparing the change in bond lengths of the PCPDT-BT cation to that of the polaron in Complex-1, using the same type of bond length analysis. The results, displayed in Fig. 4a , show how the distortion in bond length is more extended in the absence of F4-TCNQ, particularly on the right side of the polymer strand centre (bond number >14). It is gratifying to note that electron spin resonance measurements on a similar copolymer yielded a free polaron delocalized over three repeat units [40] , very close to our polaron size for the cation. The comparison between cation and Complex-1 indicates that in the latter the negatively charged F4-TCNQ molecule exerts an electrostatic attraction on the positive polaron on the polymer, contributing to confine it. The more delocalized polaron for the cation leads to a red-shift of the most intense vibrational band to 880 cm −1 ( Fig. 3a ). Signatures of this mode in experiments have not been detected, suggesting that most of the holes on the doped copolymer film remain bound to the ionized F4-TCNQ, that is, in a configuration similar to Complex-1. We obtain a similar red-shift of the low-frequency vibrational bands (from ca . 1,050 to ca . 900 cm −1 ) between the calculated spectra of Complex-3 and PCPDT cation ( Fig. 3d ), indicating that also for the homopolymer the polaron is localized by the Coulomb interaction with the negatively charged F4-TCNQ. Figure 4c illustrates with displacement vectors the vibrational mode at 1,033 cm −1 , corresponding to the most intense peak in the calculated spectrum of Complex-1 ( Fig. 3a ). Comparing Fig. 4b,c , it can be seen how the biggest atomic displacements of this mode happen to be in the region where the polaron is located. The enhancement in absorption intensity associated with this mode is consistent with previous results, which have argued that the oscillation of the polaron charge density concomitantly with a vibrational mode can result in an increase in the transition dipole moment [27] . Thus, for the case of PCPDT-BT, while the charge transfer occurs when F4-TCNQ is close to the D moiety, the bond vibrations involving the two nearest neighbours A moieties on which the polaron wavefunction delocalizes give an important contribution to the mode absorption intensity. Future experiments on charge-sensitive vibrations using infrared near-field microscopy [41] or two-dimensional coherent infrared spectroscopy [42] could provide further important insights on the mesoscopic structure and electronic couplings between dopant and adjacent polymer strands. From the materials point of view, the recently discovered doping via Lewis acids [43] , [44] offers a new interesting system where the impact of intermolecular disorder needs to be explored. In conclusion, we studied the microscopic details of the formation of hole polarons induced by the dopant molecule F4-TCNQ on the D–A copolymer PCPDT-BT, showing the crucial influence of intermolecular geometrical disorder on the efficiency of doping. By exploiting the high sensitivity of vibrational spectroscopy to the presence of charged species on the polymer chains, we have probed that polarons are formed only above a molar ratio of 4%. This concentration is rather high compared with what we observed in the homopolymer PCPDT, where the formation of polarons was observed already at 1%. These observations can explain the low doping efficiency previously shown in transport measurements on doped D–A copolymers. Here we were able to pinpoint the intermolecular factors contributing to the low doping efficiency by theoretically simulating infrared spectra. We showed that the efficiency of charge transfer from copolymer to dopant strongly depends on the intermolecular geometry. The design of new dopants with a larger molecular size bridging the entire repeat unit of copolymers could be a strategy to overcome these limitations. Materials, thin-film preparation and FTIR PCPDT-BT ( M w =34 kg mol −1 , polydispersity (PD)=2.1, purity=99.99%, based on trace metals content) was purchased from 1-Material and used as received. PCPDT ( M w =26 kg mol −1 , PD=1.8) was synthesized in a Yamamoto type polycondensation reaction of 2,6-dibromo-4,4-bis(2-ethylhexyl)-4H-cyclopenta[2,1-b:3,4-b′]dithiophene as described in the literature [45] . The molecular weight of PCPDT was measured on a PSS/Agilent SECurity GPC equipped with MZ Gel SDplus linear columns, a VWD G1329A ALS ultraviolet detector, and a RID C1362A RI detector, using chloroform as eluent. F4-TCNQ (purity ≥98%) was purchased by TCI-europe and used as received. The HOMO levels of PCPDT-BT and PCPDT were measured in film on a Riken Keiki AC-2 spectrometer. We measured the energy of the HOMO levels of PCPDT-BT and PCPDT by photoelectron spectroscopy under ambient conditions, and have obtained values with respect to vacuum of −5.07 and −5.08 eV, respectively. Therefore, we exclude that the difference in doping efficiency observed between the two polymers is owing to a difference in energetics of the two systems. For the LUMO level of F4-TCNQ, we consider the value reported in literature of −5.24 eV (ref. 46 ). Infrared spectra were recorded in transmission mode on a PerkinElmer Frontier FTIR spectrometer at room temperature. Thin-film samples for FTIR spectroscopy were fabricated by spin coating polymer and F4-TCNQ dissolved in chlorobenzene. The solutions were prepared as follows: a starting F4-TCNQ solution was prepared (0.875 mg ml −1 ) and the appropriate amount was added to a separate polymer solution to obtain the desired molar percentages. In the final solutions, the polymer concentration was always 10 mg ml −1 . The solutions were spin coated onto pre-cleaned CaF 2 substrates in nitrogen atmosphere. The optimal spin speeds for film homogeneity were found at 900 and 1,500 r.p.m. for PCPDT and PCPDT-BT, respectively. Quantum chemistry calculations Ab initio molecular orbital calculations were performed using the Gaussian 09 and Firefly suite of programs. Owing to the extremely large number of conformational degrees of freedom, great attention and a large endeavour was devoted to a detailed conformational analysis of the Complexes ( Supplementary Figs 12 and 13 , and Supplementary Discussion ). To reduce the computational cost, alkyl side chains, which are likely to be uninvolved in determining electronic structure of frontier orbitals, have been largely replaced by methyl groups. A conspicuous amount of screening optimization-geometry calculations ( Supplementary Tables 1 and 2 ), as well as Hessian analysis, were carried out. In particular, CAM-B3LYP DFT was used using 6–31G** basis sets giving the best agreement with the experimental vibrational spectra. Calculations on the PCPDT-BT:F4-TCNQ Complexes were run using both R-DFT and spin-unrestricted DFT wavefunctions. Restricted calculations (R-DFT) yield a much more limited intermolecular charge separation, resulting in a Mulliken net charge of 0.04 e on F4-TCNQ. As discussed by us [47] and other authors [22] , unrestricted calculations are more suitable for describing charge states and R-DFT was used only for control experiments ( Fig. 4a ). All the calculations were performed without any symmetry constraints (that is, C1 point group symmetry). Aiming to account for the influence of the surrounding condensed phase, the calculations were performed including electrostatic interactions between the polymer or Complex under study and a polarizable continuum medium with relative dielectric constant 3. This was done exploiting the solvation model based on density [35] as implemented in Gaussian 09. The stabilization energies for Complexes-1 and -2 are −0.46 and −0.22 eV, respectively ( Supplementary Table 1 ). For each vibrational mode, the integrated absorption intensity was calculated (units of cm mol −1 ; ref. 48 ). To better fit the experimental spectra, we introduced a broadening by multiplying each computed absorption line of wavenumber f 0 with a unitless Lorentzian-like function of the form , where a is the full-width at half-maximum. We chose to use a =15 cm −1 . Note that, in general, the computed vibrational bands, especially at higher wavenumbers, are blue shifted compared with the experimental ones. This is a well-known effect arising from the parabolic potentials used in calculating the vibrational bands [49] . To account for this, and following standard procedures, we have rescaled the wavenumber axis of the computed spectra by a factor of 0.935 for wavenumbers >1,280 cm −1 (refs 36 , 50 ). For frequencies <1,280 cm −1 , no scaling was applied. Full and unscaled spectra are shown in the Supplementary Discussion ( Supplementary Figs 14 and 15 ). How to cite this article: Di Nuzzo, D. et al . How intermolecular geometrical disorder affects the molecular doping of donor–acceptor copolymers. Nat. Commun . 6:6460 doi: 10.1038/ncomms7460 (2015).